Coherence and modality of driven interlayer-coupled magnetic vortices The high-frequency dynamics of mode-coupled magnetic vortices have generated great interest for spintronic technologies, such as spin-torque nano-oscillators. While the spectroscopic characteristics of vortex oscillators have been reported, direct imaging of driven coupled magnetic quasi-particles is essential to the fundamental understanding of the dynamics involved. Here, we present the first direct imaging study of driven interlayer coaxial vortices in the dipolar- and indirect exchange-coupled regimes. Employing in situ high-frequency excitation with Lorentz microscopy, we directly observe the steady-state orbital amplitudes in real space with sub-5 nm spatial resolution. We discuss the unique frequency response of dipolar- and exchange-coupled vortex motion, wherein mode splitting and locking demonstrates large variations in coherent motion, as well as detail the resultant orbital amplitudes. This provides critical insights of the fundamental features of collective vortex-based microwave generators, such as their steady-state amplitudes, tunability and mode-coupled motion. Magnetic-based technologies have recently garnered much attention as an alternative to traditional electronics with the potential of scalability, low-power operation and radiation hardness. Many of these proposed spintronic devices utilize magnetic solitons constrained as fundamental elements in mesoscopic and nanoscopic ferromagnetic (FM) structures. The remarkable stability of topological solitons and other highly localized nanomagnetic structures under spin currents and Oersted field excitation has not only motivated spin-based oscillator technologies, but also memories and logic devices [1] , [2] , [3] , [4] , [5] , [6] , [7] , [8] , [9] , [10] , [11] , [12] . Notably, magnetic vortices are a type of quasi-particle that possess an out-of-plane magnetization, known as the vortex core polarity P =[+,−] (up or down), and an in-plane circular magnetization surrounding the core C =[+,−] (clockwise or anti-clockwise), often referred to as the chirality [13] . The two degrees of freedom of magnetic vortices offer an intriguing opportunity to study linear and nonlinear high-frequency (HF) dynamics at room temperature, as well as to directly observe the motion of collective quasi-particle systems, which is critical for HF applications [14] , [15] , [16] . When a vortex is perturbed by a pulsed signal or sinusoidal wave near the eigenfrequency [17] , [18] , HF excitations are generated as a result of the translational motion of the core. Indeed, utilizing such perturbations has demonstrated excellent linewidths with frequencies in the gigahertz range, and device compatible power generation using phase-locked vortices in carefully engineered geometries and materials [19] , [20] . Recently, the use of interlayer-coupled (IC) solitons in multilayered structures has resulted in higher velocities, the reversal of magnetic ordering through ion irradiation, as well as independent control of the vortices’ polarity and chirality in heterostructures with polarized spin currents [21] , [22] , [23] . To the best of our knowledge, the direct observation of HF dynamic motion in coaxial strongly coupled vortex system has yet to be reported and will provide significant insights for applications such as spin-torque vortex oscillators (STVO). The performance metrics of STVOs, such as power output and spectral linewidths, are directly related to the vortex core rigidity, coherent gyrotropic motion, steady-state orbital amplitude and mode-coupled dynamics [1] , [2] , [12] , [19] , [24] , [25] . Here we present a direct imaging study of the driven dynamics in IC magnetic vortex disc heterostructures. We report on the existence and coherence of the collective modes, the variations of the orbital amplitudes due to local structure and the frequency response of magnetostatic and indirect exchange-coupled (IEC) spin vortex oscillators. The results provide an experimental foundation for studying more complex systems where three-dimensional (3D) nanowires of n -vortices’ stacks could be used to generate enhanced HF signals compared with their single-layered counterparts [26] , [27] . In a thin FM disc, the demagnetization energy serves as a restorative force for the vortex core, and ordinary gyrotropic precessional dynamics can be captured using a harmonic oscillator model [28] . As the core precesses, magnetic charges form on the edges of the disc and stray fields associated with these charges have been used to laterally couple neighbouring vortices [17] , [29] , [30] . These magnetostatic interactions are long range but weak, and even edge-overlapped direct exchange discs may demonstrate complex nonlinearities [15] . Alternatively, a stacked geometry increases the magnetic interaction over the entire surface of the FM layers, thus leading to strong coupling of coaxially aligned vortices. 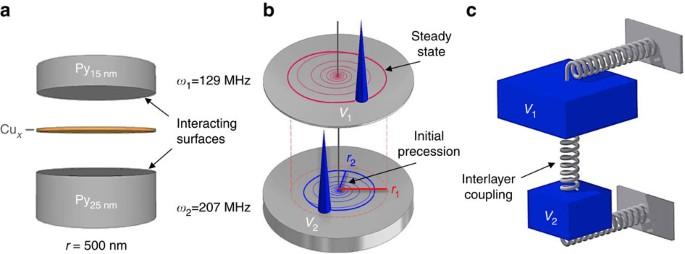Figure 1: Coaxial vortex systems. (a) A diagram of a multilayered structure, wherein the thickness of the Cu spacer layer is varied to change the strength of the interaction between the two FM layers. (b) The dissimilar gyrotropic motion of the vortex cores (V1,V2) at the respective eigenfrequencies (ω1<ω2) is due to the asymmetry in thickness of the isolated FM layers. After the initial precessional motion, the applied sinusoidal field at the primary eigenfrequency drives the steady-state dynamics, and although the same field magnitude is applied to both discs, the asymmetry results in dissimilar orbital amplitudes (r1>r2). (c) The cores contained within each layer in the stack can be treated as harmonic oscillators where the Cu spacer layer provides an interlayer coupling energy represented by an additional spring coupling the two masses. The strength of the interlayer coupling depends on the thickness of the Cu spacer layer, allowing short-range exchange and long-range magnetostatic interactions. Figure 1a shows an exploded diagram of the heterostructures fabricated in this work, where the thicknesses of the two FM layers were fixed at 25 and 15 nm of permalloy (Py), separated by a thin Cu layer. At rest, a vortex core resides in the centre of the disc, which is the energy minimum of the potential. If the two FM layers of the device are isolated and excited with a HF field at resonance, the orbital amplitude of the steady-state vortex core-path trace ( r 1 , r 2 ) as well as the eigenfrequency ( ω 1 , ω 2 ) are distinct as shown in Fig. 1b . The vortices can be interpreted as two harmonic oscillators, as shown in Fig. 1c , with dissimilar restorative spring constants and masses due to the thickness asymmetry. The non-magnetic (NM) Cu layer provides a means of coupling the two vortices and can be understood as a spring coupling the two masses together. Both magnetostatic and indirect exchange-coupling regimes were investigated by varying the thickness of the NM spacer with angstrom-level accuracy. We discuss the role of interlayer coupling and different excitation modes, wherein the two vortices could exhibit coupled modes, such as acoustic and optical [29] , [31] , or, if the coupling is weak, independent gyrotropic motion. The asymmetry in the FM layers was chosen to exploit the non-overlapping eigenmodes, which become more evident in the frequency spectrum under weak coupling, and can serve to independently control the states of the vortices. To promote coherent oscillations, we initialized all the vortices to similar polarities and chiralities ( P 1 , P 2 )=[+, +], ( C 1 , C 2 )=[+, +]. Figure 1: Coaxial vortex systems. ( a ) A diagram of a multilayered structure, wherein the thickness of the Cu spacer layer is varied to change the strength of the interaction between the two FM layers. ( b ) The dissimilar gyrotropic motion of the vortex cores ( V 1 , V 2 ) at the respective eigenfrequencies ( ω 1 < ω 2 ) is due to the asymmetry in thickness of the isolated FM layers. After the initial precessional motion, the applied sinusoidal field at the primary eigenfrequency drives the steady-state dynamics, and although the same field magnitude is applied to both discs, the asymmetry results in dissimilar orbital amplitudes ( r 1 > r 2 ). ( c ) The cores contained within each layer in the stack can be treated as harmonic oscillators where the Cu spacer layer provides an interlayer coupling energy represented by an additional spring coupling the two masses. The strength of the interlayer coupling depends on the thickness of the Cu spacer layer, allowing short-range exchange and long-range magnetostatic interactions. Full size image Determination of resonance for strongly interlayered coupled vortices Unpatterned thin-film multilayers were characterized using FM resonance (FMR) to determine material parameters, such as magnetic saturation and damping ( Supplementary Fig. 1 ). To extract the effective IEC energy, the NM Cu spacer layer was varied while maintaining the 15 and 25 nm Py FM layer thicknesses. A Cu spacer layer thickness of 1 nm was determined to possess strong effective IEC, and the film continuity was verified via atomic force microscopy to ensure that unintended direct Heisenberg exchange interactions were avoided ( Supplementary Fig. 2 ). The 3D micromagnetic simulations were implemented using the extracted values from the FMR experiments to clarify the dynamic nature of coupled vortex oscillations near gigahertz frequencies. The precessional eigenfrequencies of single-layered discs were calculated using both an analytical model and micromagnetic simulations for various thicknesses and radii as shown in Fig. 2 . 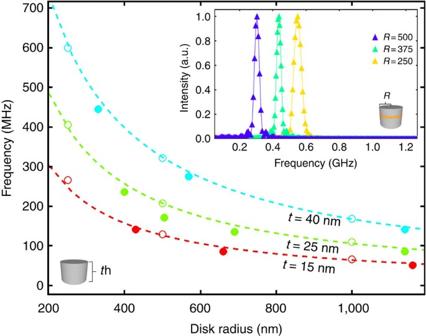Figure 2: Eigenmodes of vortex systems. Eigenfrequencies of single-layered discs where the red, green and light blue represent thicknesses of 15, 25 and 40 nm over various radii. Micromagnetic, analytical and experimental values are given, respectively, by the open markers, dotted lines and solid markers. The inset shows the Fourier transformation of the numerically simulated frequency spectra for Py25 nm|Cu1 nm|Py15 nmmultilayered discs, wherein the blue, green and gold plots are 500, 375 and 250 nm in radius. The fundamental mode is represented by the peak in the spectra, and the absence of any further harmonics indicates that the two cores in the multilayered discs are mode coupled. The analytical model used to calculate the eigenfrequencies was a side-charge-free model [32] , Figure 2: Eigenmodes of vortex systems. Eigenfrequencies of single-layered discs where the red, green and light blue represent thicknesses of 15, 25 and 40 nm over various radii. Micromagnetic, analytical and experimental values are given, respectively, by the open markers, dotted lines and solid markers. The inset shows the Fourier transformation of the numerically simulated frequency spectra for Py 25 nm |Cu 1 nm |Py 15 nm multilayered discs, wherein the blue, green and gold plots are 500, 375 and 250 nm in radius. The fundamental mode is represented by the peak in the spectra, and the absence of any further harmonics indicates that the two cores in the multilayered discs are mode coupled. Full size image where γ is the gyromagnetic constant, M s is the magnetic saturation, E l is the exchange length, R is the disc radius and F v ( β ) is a function of the disc’s aspect ratio β . The analytical calculations are represented by the dotted lines, the open circles are the micromagnetic simulations and the solid circles are the experimentally determined eigenfrequency using Lorentz microscopy. The red, green and blue colours represent 15, 25 and 40 nm single-layered vortex disc thicknesses, respectively. We note that the 15 and 25 nm thicknesses are the bottom and top layer of the multilayer stack, and therefore, the summation of these two layers should be comparable to a single-layered 40 nm disc. Interestingly, the 40-nm-thick single-layered discs did not act as an upper bound of the eigenfrequencies and the IEC heterostructures exhibited slightly higher resonance, as discussed in the experimental section. To determine the eigenfrequencies of the asymmetric disc heterostructures, we ran micromagnetic simulations using a two-surface exchange energy implemented across the 1-nm Cu spacer layer [33] . The 3D structure was perturbed by a small static field, and the magnetic evolution was solved by a Runge–Kutta approximation of the ordinary differential Landau–Lifshitz–Gilbert equation, where γ G is the Gilbert gyromagnetic ratio, is the summation of the demagnetization field, Zeeman Field, exchange interaction, and anisotropy, is the magnetization and α is the damping constant. For reasonable simulation times, the largest simulated radius of the multilayer disc was 500 nm. The inset of Fig. 2 is a Fourier transformation of the vortex cores’ periodic motion during relaxation after perturbation for 250, 375 and 500 nm multilayered disc radii. As is evident in the simulated frequency domain, each disc had a singular peak in the sub-gigahertz range; no higher harmonics of the primary modes were detected up to 10 GHz. This specifies a surface exchange interaction energy of 1 × 10 −3 J m −2 ( Supplementary Fig. 1 ) for a 1-nm-thick Cu spacer layer should mode-lock the two vortices into a singular eigenmode. TEM measurements of the collective dynamics The ultra-high resolution magnetic imaging capabilities (<5 nm) of Lorentz transmission electron microscope (LTEM), combined with a uniquely designed objective lens [34] and custom HF sampler holder used in this work, enabled detailed observations of the coupled vortex dynamics. 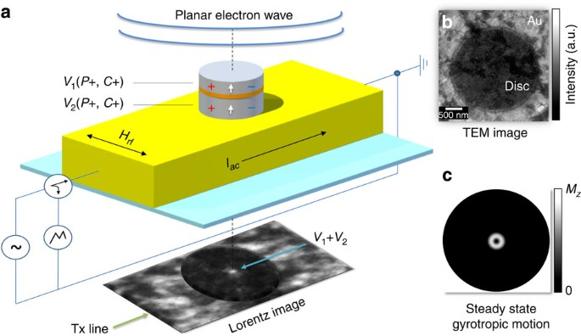Figure 3: Device schematic and TEM imaging. (a) A schematic of the patterned heterostructure containing two magnetic vortex cores on top of an Au waveguide and Si3Ni4membrane (not to scale). Lorentz TEM records the projected in-plane magnetization over the entire thickness of the multilayer stack, and simultaneously captures both vortex cores. The magnetic chirality of the two FM-coupled vortex structures cause the beam to converge, producing a central bright spot. (b) An in-focus TEM image of the disc on top of the polycrystalline Au waveguide. (c) Micromagnetic simulations of the magnetization averaged over the thickness of a single layer–single vortex disc under HF excitation. The gyrotropic orbit found in the central region of the disc reflects the periodic oscillations of a single vortex core in response to the applied HF Oersted field averaged over 2 ns. Figure 3a is a schematic of the device with an electrical circuit diagram. The device was driven by a signal generator that provided a sinusoidal waveform from 100 KHz up to 1 GHz. The signal was passed through a directional coupler that then fed into the waveguide shown in Fig. 3a , as well as a HF oscilloscope. The vortex discs were fabricated on Au waveguides and Si 3 N 4 support membranes. Below the schematic is an LTEM image that details the multilayered disc and Au transmission line that provided the HF excitation via an Oersted field. The in-plane magnetic contrast of LTEM was observed under a defocused beam condition [35] and is sensitive to the magnetic vortex configuration in both layers simultaneously [36] . The bright spot in the centre of the disc in Fig. 3a is the magnetic structure caused by both vortex cores at rest. Figure 3b is an in-focus TEM image of the device where the background is the polycrystalline grains of the Au waveguide and the disc heterostructure is in the foreground. When excited by a HF signal at the respective primary eigenfrequency, an ordinary single vortex core will reach a steady-state precessional motion [37] . The trace of the time-averaged steady-state single vortex’s core path generates a ring-like contrast of the vortex’s orbit (abstracted in Fig. 1b ), which is simulated and averaged for over 2 ns in Fig. 3c . The orbit’s radial amplitude is a function of the external stimulus and the disc’s properties, such as shape and crystalline anisotropy. The brighter intensity reflects the repeated spatial presence of the vortex core (that is, the out-of-plane magnetization M z ) integrated over time, precessing away from equilibrium. The darker areas, such as the in the central region where the core would reside at rest, represent the absence of the vortex, and hence the consequent lack of intensity. Accordingly, we can address the question of whether multiple vortices can have collective modes and be directly imaged. If two cores are weakly coupled, then the frequency spectrum should exhibit two resonant modes, corresponding to the eigenfrequencies of the individual layers. On the other hand, using a thin spacer layer can introduce indirect exchange interactions between the two vortices over the FM surfaces ( Fig. 1a ), as well as strong magnetostatic interactions. If this coupling is sufficiently robust, our micromagnetic simulations suggest that there is a single eigenmode in the frequency spectrum corresponding to the mode-coupled oscillations. Figure 3: Device schematic and TEM imaging. ( a ) A schematic of the patterned heterostructure containing two magnetic vortex cores on top of an Au waveguide and Si 3 Ni 4 membrane (not to scale). Lorentz TEM records the projected in-plane magnetization over the entire thickness of the multilayer stack, and simultaneously captures both vortex cores. The magnetic chirality of the two FM-coupled vortex structures cause the beam to converge, producing a central bright spot. ( b ) An in-focus TEM image of the disc on top of the polycrystalline Au waveguide. ( c ) Micromagnetic simulations of the magnetization averaged over the thickness of a single layer–single vortex disc under HF excitation. The gyrotropic orbit found in the central region of the disc reflects the periodic oscillations of a single vortex core in response to the applied HF Oersted field averaged over 2 ns. 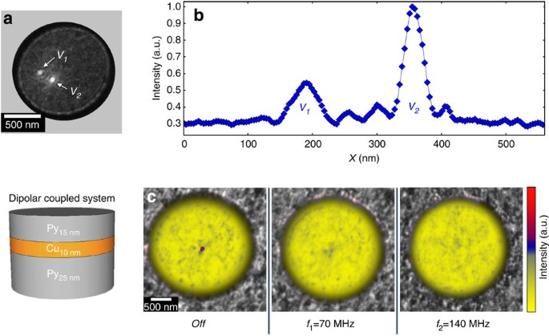Figure 4: Dipolar-coupled vortices. (a) An LTEM image of a disc heterostructure with a 10 nm NM spacer Cu layer under a quasi-static perturbation. The two cores are labelled (V1,V2) and correspond to the top and bottom layers, respectively. (b) A line scan through both cores where the intensity verifies the thickness asymmetry between the two FM layers and corresponding magnetic contrast. (c) A series of LTEM images depict three situations (colour enhanced to accentuate magnetic contrast), where the applied field is off, the applied field frequency isf1=70 MHz andf2=140 MHz. The two vortex cores are captured simultaneously and can be seen overlapping at the equilibrium position with the field off. The frequency was swept from 100 kHz to 1 GHz and atf1andf2the contrast from the vortices is no longer present due to decoherent motion. Full size image Mode splitting of dipolar-coupled vortices Figure 4 shows experimental results for a representative disc heterostructures with a 10-nm-thick NM Cu spacer layer. From our FMR experiments ( Supplementary Fig. 1 ), the indirect exchange interaction for our multilayered films approached zero for thickness above 2 nm. Therefore, in these systems the contribution from indirect exchange interactions can be neglected and only magnetostatic interactions can account for the coupling of the two vortices in the top and bottom FM layers. The full-field imaging of LTEM simultaneously captures the magnetization of the entire disc, and in Fig. 4a , an in-plane quasi-static applied field was used to perturb the vortices into a non-overlapping state. Figure 4b is a line scan of V 1 and V 2 and shows the variation in intensity due to the thickness asymmetry found in the FM layers. The system shown in Fig. 4c was not perturbed by an applied in-plane quasi-static field and the cores are superimposed in the equilibrium position (red central peak). The colour enhancement was used to accentuate the magnetic contrast in the HF LTEM experiments. For the frequency sweep (100 kHz to 1 GHz) in Fig. 4c , minimal broadening of the vortices’ peak was detected, except for the two cases depicted, at f 1 =70 MHz and f 2 =140 MHz. These two frequencies are near the expected single-layered eigenfrequencies (see Fig. 2 ), which suggest that the top and bottom layers were excited near their respective isolated eigenfrequencies. Figure 4: Dipolar-coupled vortices. ( a ) An LTEM image of a disc heterostructure with a 10 nm NM spacer Cu layer under a quasi-static perturbation. The two cores are labelled ( V 1 , V 2 ) and correspond to the top and bottom layers, respectively. ( b ) A line scan through both cores where the intensity verifies the thickness asymmetry between the two FM layers and corresponding magnetic contrast. ( c ) A series of LTEM images depict three situations (colour enhanced to accentuate magnetic contrast), where the applied field is off, the applied field frequency is f 1 =70 MHz and f 2 =140 MHz. The two vortex cores are captured simultaneously and can be seen overlapping at the equilibrium position with the field off. The frequency was swept from 100 kHz to 1 GHz and at f 1 and f 2 the contrast from the vortices is no longer present due to decoherent motion. Full size image A distinctive feature of the dipolar-coupled heterostructure shown in Fig. 4 , when compared with the respective isolated single layers, is the interaction between the two vortex core results in the loss of contrast near f 1 and f 2 . As depicted in Fig. 3c , when a single vortex core is isolated and excited at the eigenfrequency, the time-averaged motion yields a steady-state orbit from the periodic motion. However, the LTEM images of Fig. 4c at f 1 and f 2 revealed no such contrast suggestive of non-trivial magnetostatic interactions that may destabilize the orbit. Indeed, since they are not isolated, when the core of the thicker bottom layer is excited it interacts with the vortex of the thinner top layer through dipolar fields, and vice versa. The LTEM images clearly show an absence of any static or highly coherent periodic motion. The lack of steady-state motion is interesting and could have several explanations, such as nonlinear interactions where, for example, the cores may reach critical velocities and reverse polarities [15] , [38] , [39] , [40] , [41] , [42] . This clearly demonstrates that while the dipolar-coupled systems we present here still respond at characteristic frequencies, the collective modes can be convoluted and require further care when describing the resultant coupled vortex motion. Mode-locked IEC vortices To establish coherent oscillations of coupled vortex disc heterostructures, the spacer thickness was reduced to 1 nm as shown in Fig. 5 . This introduced a stronger coupling through an indirect exchange interaction across the inner boundary surfaces of the FM layers ( Fig. 1a ). 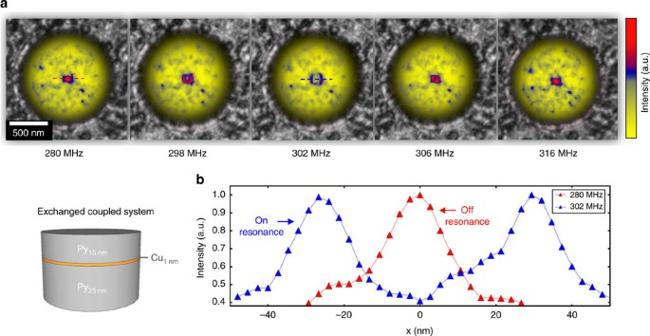Figure 5: IEC vortices. (a) LTEM images of multilayered disc (r≈500 nm) throughout a frequency sweep (colour enhanced to accentuate magnetic contrast). The singular orbit near resonance of the multilayer disc demonstrates the spatial coherence of the two vortices’ gyrotropic motion, which is also supported by micromagnetic simulations. (b) Line scans of the Lorentz TEM images off resonance at 280 MHz (red) and on resonance at 302 MHz (blue). The off resonance scan shows a single peak where the two vortices are directly on top of one another. Interestingly, when excited at resonance, a singular gyrotropic orbit appears as shown by the two peaks at 302 MHz. If one of the vortex cores was decoupled from the steady-state motion, we should detect the other magnetic contrast. Instead, a local minimum of magnetic contrast was observed at the centre of the disc (where both cores reside at rest), with a highly coherent gyrotropic orbit, and no additional magnetic contrast. This suggests spatially coherent steady-state motion of the two strongly coupled vortices. Figure 5a shows a HF field sweep near the eigenfrequency of 302 MHz for a representative 1 μm disc. In the series of LTEM images, the orbital amplitude changes dramatically, ~60 nm in diameter, over a narrow frequency range of ±4 MHz (see Supplementary Movie 1 for more details). Even more interesting is the two cores’ periodic motion appears to be spatially coherent under the driven excitation. Figure 5b shows normalized line scans over the centre of the coupled vortex heterostructure, off resonance at 280 MHz and on resonance at 302 MHz. When excited under the former conditions, the singular peak contains both vortex cores, since LTEM is sensitive to the integrated magnetization over the entire thickness of the disc. The on-resonance line scan of the collective vortex motion at 302 MHz has two peaks signifying the increased contrast from the steady-state orbit. Unlike the dipolar-coupled discs, coherent gyrotropic motion was observed but only one orbit was detected. This suggests that the resultant effect from the indirect exchange and dipolar interactions of the two FM layers is the spatially overlapping gyrations of the two vortex cores, measured in a singular time-averaged orbit. Figure 5: IEC vortices. ( a ) LTEM images of multilayered disc ( r ≈500 nm) throughout a frequency sweep (colour enhanced to accentuate magnetic contrast). The singular orbit near resonance of the multilayer disc demonstrates the spatial coherence of the two vortices’ gyrotropic motion, which is also supported by micromagnetic simulations. ( b ) Line scans of the Lorentz TEM images off resonance at 280 MHz (red) and on resonance at 302 MHz (blue). The off resonance scan shows a single peak where the two vortices are directly on top of one another. Interestingly, when excited at resonance, a singular gyrotropic orbit appears as shown by the two peaks at 302 MHz. If one of the vortex cores was decoupled from the steady-state motion, we should detect the other magnetic contrast. Instead, a local minimum of magnetic contrast was observed at the centre of the disc (where both cores reside at rest), with a highly coherent gyrotropic orbit, and no additional magnetic contrast. This suggests spatially coherent steady-state motion of the two strongly coupled vortices. Full size image To support the mode-locked spatially coherent motion observed in the IEC systems, the LTEM orbital amplitude was measured as a function of the excitation frequency for different disc radii in Fig. 6a . The HF field was scanned from 100 kHz to 1 GHz for numerous elements. As depicted by the fitted curves, the peak orbital amplitude scales as a function of the disc’s radius due to the increased demagnetization energy as the core moves closer to the edges of the disc, and occurs at the eigenfrequency. Figure 2 plots the experimentally determined eigenfrequency for single vortex discs of different thicknesses, and clearly shows the distinct eigenfrequency at any specific radius. This is an important consideration given the 15 and 25 nm thicknesses, respectively, comprise the bottom and top layers of the heterostructures. While sweeping the frequency for IEC discs of radii ranging from ~300–1,000 nm, all the discs demonstrated a single eigenfrequency with no mode splitting (in contrast to the purely dipolar-coupled discs). The single orbit observed at resonance combined with the unique eigenfrequency found in these IEC discs strongly supports mode-locked gyrotropic motion of the two vortex cores. To further distinguish the coherent gyrotropic motion of the IEC vortex discs, we considered the steady-state motion of comparable single vortex systems. 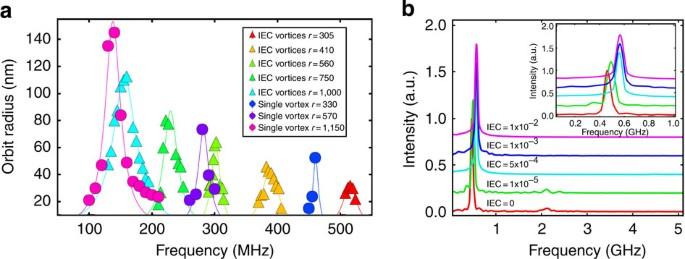Figure 6: The effects of IEC on strongly coupled vortices. (a) The solid circles are experimental values for the spatially coherent orbits of the single-layered vortex discs with radii ranging from 305 to 1,000 nm. The eigenfrequency was defined for each disc as the maximum orbital amplitude of the core gyration, and therefore, the fitted curves’ peak positions. The solid triangles are the comparable IEC vortex discs. The effect of the 1-nm Cu bifurcation compared with that of the single vortex disc was an upward shift in the resonance frequency. The reduction in the overall amplitude of the orbits was attributed to variations in the strength of the applied field. The singular eigenmode for the two-vortex systems supports our conclusion of spatially coherent oscillations. (b) Normalized Fourier transformation of the finite-element simulations for Py25nm|Cu1nm|Py15nmwhere the IEC was varied forr=250 nm, and the lines are shifted in theydirection by 0.20 for presentation purposes. When the IEC is negligible, a primary collective mode is present near 0.5 GHz and another secondary mode at 2.1 GHz. As the IEC value approaches physically meaningful values (~1 × 10−3J m−2), the secondary mode is quenched and primary mode, detailed in the inset, is shifted upward. Figure 6: The effects of IEC on strongly coupled vortices. ( a ) The solid circles are experimental values for the spatially coherent orbits of the single-layered vortex discs with radii ranging from 305 to 1,000 nm. The eigenfrequency was defined for each disc as the maximum orbital amplitude of the core gyration, and therefore, the fitted curves’ peak positions. The solid triangles are the comparable IEC vortex discs. The effect of the 1-nm Cu bifurcation compared with that of the single vortex disc was an upward shift in the resonance frequency. The reduction in the overall amplitude of the orbits was attributed to variations in the strength of the applied field. The singular eigenmode for the two-vortex systems supports our conclusion of spatially coherent oscillations. ( b ) Normalized Fourier transformation of the finite-element simulations for Py 25nm |Cu 1nm |Py 15nm where the IEC was varied for r =250 nm, and the lines are shifted in the y direction by 0.20 for presentation purposes. When the IEC is negligible, a primary collective mode is present near 0.5 GHz and another secondary mode at 2.1 GHz. As the IEC value approaches physically meaningful values (~1 × 10 −3 J m −2 ), the secondary mode is quenched and primary mode, detailed in the inset, is shifted upward. Full size image The frequency spectra in Fig. 6a are characteristic LTEM measurements of the time-averaged orbital amplitudes for IEC discs, as well as for equivalent single-layered discs (that is, 40 nm thick). Since we measured the real-space gyrotropic motion for individual discs with sub-5 nm resolution, the data points are directly related to the vortices’ response to the HF excitation and local structure. The deviations of the measured orbital amplitudes from the fitted Lorentzian curves are unique to each disc and are related to the inherent microstructure [43] . For example, the asymmetry of the data for the single vortex disc r =1150, nm demonstrates good agreement with the fit in the onset of the curve but a more linear trend towards the end where the orbital amplitude tails off. The ability to measure the steady-state orbit with such high fidelity demonstrates the effects of the inherent structure on the vortex’s dynamics by retarding the expansion or collapse of the orbit of the highly localized magnetic quasi-particle. This is important when considering the similar geometries of STVOs, which also could be susceptible to similar spectral broadening and narrowing due to local defects. Comparing the maximum orbital amplitudes of the single vortex systems reveals that they tend to be slightly larger than the IEC vortices; we attribute this to the single vortex and dual vortex systems being on different coplanar waveguides (that is, different applied field strengths). However, in comparison to the single layers, the blue shifts of the IEC disc’s eigenfrequencies are not as sensitive to slight variations of the applied field strength. These frequency shifts were observed for all the discs and we attribute this to the non-overlapping eigenmodes in the two distinct FM layers synchronized through exchange coupling. The effects of coupling on collective dynamics To understand the role of dipolar and indirect exchange coupling on interacting vortices, numerical simulations were undertaken of a disc heterostructure for r =250 nm, a Cu layer thickness of 1 nm and varying IEC constants as shown in Fig. 6b . When the IEC values are near zero, a primary mode (~0.5 GHz) and secondary mode (~2.1 GHz) are present in the frequency domain. These are collective modes, which are higher than the isolated eigenfrequencies of either the top or bottom discs ( Fig. 2 ), and result from dipolar coupling. As the IEC is increased, the secondary mode is quenched and the primary mode is shifted upward by ~20% for physically meaningful IEC values. The blue shift of the primary mode for IEC energy near the experimental values of 5 × 10 −3 , 1 × 10 −3 and 1 × 10 −2 J m −2 are much narrower at 559, 562 and 565 MHz, respectively, and show good agreement with the LTEM experimental trends illustrated in Fig. 6a . This establishes another degree of resonant frequency tunability through modifying the coupling strength and eigenfrequencies of the individual discs. We also note that when the thickness of a single-layered vortex disc reaches a critical aspect ratio (thickness to radius), the core becomes non-rigid [2] , and eventually, transitions into an energetically favourable single-domain state as found in nanowires. Therefore, the aspect ratio of single-layered discs is limited to quasi-2D elements for applications that require a rigid vortex core for coherent oscillations. By using IEC disc heterostructures, these transitions can be mitigated by the physical boundaries of NM spacer layers between the vortex layers, while maintaining mode-locked oscillations through indirect exchange interactions ( Fig. 5 ). Using coaxially aligned vortex disc heterostructures, we investigated the effects of dipolar and indirect exchange interactions on driven collective dynamics. Dipolar-coupled heterostructures (Cu 10 nm ) demonstrated mode splitting that was determined by variances in the LTEM magnetic contrast near the non-overlapping eigenfrequencies of the equivalent isolated single-layered vortex discs. For IEC discs (Cu 1 nm ), we detected spatially coherent gyrotropic motion of mode-locked vortices with a singular eigenfrequency due to the IEC. Our direct observations of strongly coupled coaxial vortex motion demonstrates that while coupled vortices may exhibit a frequency response, their resultant motion are not equally coherent. This is critical for vortex spin-wave technologies whose essential features, such as linewidths, frequency agility and power [24] , are directly related to highly coherent gyrotropic motion and orbital amplitudes [12] , [25] . Compared with single vortex- and dipolar-coupled discs, exchange-coupled vortex discs possess a higher resonance, so adding another means of tuning the eigenfrequency through strong coupling interactions. These IC vortex structures show promise for synchronizing multi-vortex nanowires for HF applications, such as spin-based antenna arrays, and our findings suggest that highly coherent gyrotropic motion will be directly related to the coupling strength between the discs. Fabrication and experimental setup The thin films were deposited in a custom ultra-high vacuum co-evaporation chamber in the department of CMPMS, BNL. The disc dimensions were chosen to nucleate magnetic vortices. The polarity of the vortices were set by saturating the structures with an out-of-plane field of over 1 T, during which we were able to resolve the annihilation of the vortex states. The field was gradually removed, using the Zeeman interaction to promote the polarity of the cores along the field direction, and was corroborated with micromagnetic simulations. The chiralities were determined via LTEM, which is directly sensitive to the in-plane magnetization [35] . The FMR spectrum of the thin films was acquired under various field strengths employing a coplanar waveguide and vector network analyzer at the NSLS, BNL. The disc heterostructures were fabricated using an electron beam lithography and liftoff process at the CFN, BNL, with a FEI Helios dual-beam system. A Veeco Multimode V scanning probe microscope was utilized to observe the surface morphology as well as film thickness of the spacer layers. The experiments were carried out in situ with a custom-built HF sample holder in a specially designed JEOL 2100F-LM TEM with a near-zero Oersted remanent field in the department of CMPMS, BNL. Micromagnetic simulations Simulations were implemented on a linux cluster in the CMPMS Department, BNL. The NIST provided Object-Oriented Micromagnetic Framework (OOMMF) Oxsii solver [33] was used in a non-uniform memory architecture to simulate the 3D disc heterostructures with a cell size of 5 × 5 × 1 nm 3 . Simulation parameters were extracted from the thin-film FMR data, where Ms=800 kA m −1 , α =0.01 and IEC 1 nm =1 × 10 −3 J m −2 . How to cite this article: Pulecio, J. F. et al . Coherence and modality of driven interlayer-coupled magnetic vortices. Nat. Commun. 5:3760 doi: 10.1038/ncomms4760 (2014).